Critical role of histone demethylase Jmjd3 in the regulation of CD4+T-cell differentiation Epigenetic factors have been implicated in the regulation of CD4 + T-cell differentiation. Jmjd3 plays a role in many biological processes, but its in vivo function in T-cell differentiation remains unknown. Here we report that Jmjd3 ablation promotes CD4 + T-cell differentiation into Th2 and Th17 cells in the small intestine and colon, and inhibits T-cell differentiation into Th1 cells under different cytokine-polarizing conditions and in a Th1-dependent colitis model. Jmjd3 deficiency also restrains the plasticity of the conversion of Th2, Th17 or Treg cells to Th1 cells. The skewing of T-cell differentiation is concomitant with changes in the expression of key transcription factors and cytokines. H3K27me3 and H3K4me3 levels in Jmjd3 -deficient cells are correlated with altered gene expression through interactions with specific transcription factors. Our results identify Jmjd3 as an epigenetic factor in T-cell differentiation via changes in histone methylation and target gene expression. CD4 + T cells consist of several subsets, including Th1, Th2, Th17 and regulatory T (Treg) cells. Th1 cells secrete interleukin (IL)-2 and interferon (IFN)-γ and express T-bet transcriptional factor, whereas Th2 cells secrete IL-4, IL-5 and IL-13, express GATA-3 and activate B cells to become antibody-secreting plasma cells [1] , [2] . Th17 cells are a distinct CD4 + Th cell lineage, secreting a unique set of cytokines including IL-17, IL-21 and IL-22 (refs 3 , 4 ). Th17 cell development and differentiation require the key transcriptional factors, retinoic acid-related orphan receptor (ROR)γt and RORα [5] , [6] . Treg cells, which express the master transcriptional regulator Foxp3, suppress host immune responses and induce self-tolerance [7] , [8] . A growing body of evidence suggests that CD4 + Th cells play a central role in initiating and maintaining immune responses against cancer and infectious and autoimmune diseases [8] , [9] , [10] , [11] . Dysregulation of CD4 + T-cell differentiation is associated with various autoimmune and inflammatory diseases, including myelodysplastic syndromes and systemic lupus erythematosus [12] , [13] , [14] . Regulation of CD4 + T-cell differentiation is essential to maintain the appropriate balance among CD4 + T-cell subsets to support immune homeostasis and prevent autoimmunity. Therefore, understanding the mechanisms regulating and controlling CD4 + T-cell differentiation into various subsets is of critical importance to develop innovative treatments. CD4 + T-subset differentiation is tightly regulated by many signalling molecules, including signal transducer and activator of transcription (STAT) proteins, IFN regulatory factor 4 (IRF4) and runt-related transcription factor 1 (refs 2 , 15 ). In addition to transcription factors, recent studies have shown that epigenetic factors control the specificity and plasticity of T-cell subsets [16] , [17] , [18] , [19] . These transcriptional factors and epigenetic regulators bind to both shared and cell-specific regulatory regions (promoters and enhancers) among various T-cell lineages and thereby, positively or negatively regulate gene expression depending upon the cofactors present [20] . It is well-known that gene expression is epigenetically regulated through DNA methylation and covalent chromatin modifications, such as histone acetylation, phosphorylation, ubiquitination, sumoylation and methylation. Histone methylation state is dynamically regulated by histone methyltransferases and demethylases [21] , [22] , [23] , [24] , [25] . Trimethylation of histone 3 at lysine 4 (H3K4) is usually associated with gene activation, whereas trimethylation of histone 3 at lysine 27 (H3K27) is associated with gene repression [21] , [22] , [23] , [24] , [25] . Polycomb repressive complex 2, containing the H3K27 methyltransferase, Ezh2, dimethylates and trimethylates H3K27 (H3K27me2/3) [24] , [26] . Recently, the H3K27 demethylase Jmjd3 (also known as KDM6B) was found to catalyse the demethylation of H3K27me2/3 in vitro [27] , [28] , [29] , [30] , [31] , [32] . Jmjd3 is induced by vitamin D and proinflammatory stimuli in macrophages and is required for Ink4a - Arf , Nodal and Irf4 expression in fibroblasts, mouse embryonic stem cells and macrophages, respectively [33] , [34] , [35] , [36] , [37] . In addition, Jmjd3 regulates macrophage differentiation, in particular, type 2 macrophages [37] , [38] . Although Jmjd3 has been shown to interact with the Th1 master regulator, T-bet [39] , [40] , the in vivo function of Jmjd3 in T-cell differentiation remains unknown. In this study, we generated T cell-specific Jmjd3 -deficient mice and found that Jmjd3 deletion promotes Th2 and Th17 differentiation and inhibits Th1 and Treg cell differentiation. Our findings indicate that Jmjd3 regulates CD4 + T-cell differentiation by mediating the methylation status of H3K27 and/or H3K4 in target genes and regulating target gene expression. These loci-specific effects of Jmjd3 on target gene expression are mediated through interactions with specific transcription and epigenetic factors. Generation of mice with T cell-specific deletion of Jmjd3 To determine the physiological role of Jmjd3 in T cells, we generated T cell-specific Jmjd3 -deficient ( Jmjd3 cKO) mice. We generated Jmjd3 flox/flox ( Jmjd3 f/f ) mice by targeting exons 15–21 (encoding the JmjC-catalytic domain) using a Cre-LoxP system [41] . Jmjd3 f/f mice were crossed with CD4-Cre mice to generate Jmjd3 cKO mice ( Supplementary Fig. 1a ). Jmjd3 cKO mice were genotyped by PCR analysis ( Supplementary Fig. 1b ). Reverse transcription (RT)–PCR and western blot analyses confirmed the loss of Jmjd3 mRNA and protein in Jmjd3 -deficient T cells, but not in B cells ( Supplementary Fig. 1c,d ). Jmjd3 cKO mice survived and grew normally. Jmjd3 skews T-cell differentiation in vivo Recent studies have shown that Jmjd3 interacts with T-bet, a master transcription factor in Th1 cell differentiation, in a histone demethylase activity-independent manner [39] , [40] . However, the in vivo function of Jmjd3 in T-cell differentiation remains unknown. To address this, we used fluorescence-activated cell sorting (FACS) analysis to determine the percentages of CD4 + T-cell subsets in lymphocytes isolated from small intestine, spleen, lymph node (LN) and colon of wild-type (WT) and Jmjd3 cKO mice. Compared with WT mice, IFN-γ-producing Th1 cells were slightly increased in the LN and colon in Jmjd3 cKO mice, but decreased in the small intestine and spleen. IL-4-producing Th2 cells were increased in the small intestine and colon, but not significantly changed in spleen or LN ( Fig. 1a–d ). The percentage of IL-17-producing Th17 cells was substantially higher in the small intestines of Jmjd3 cKO mice compared with WT mice (14.8% versus 3.8%) and in the colons (17.5% versus 5.2%) of Jmjd3 cKO mice compared with WT mice ( Fig. 1a,d ). We did not observe any appreciable changes in lymphatic Th17 cells between WT and Jmjd3 cKO mice ( Fig. 1c ). Foxp3-expressing Treg cells were slightly higher in the small intestine, spleen and LN ( Fig. 1a–c ), but not in the colon of Jmjd3 cKO mice compared with WT mice. To determine the effects of Jmjd3 on thymic and splenic natural Treg (nTreg) cell populations, WT and Jmjd3 cKO Foxp3-GFP reporter mice were generated. FACS analysis revealed that the percentage of thymic GFP + nTreg cells was approximately 50% lower in Jmjd3 cKO mice than in WT mice. In contrast, the splenic nTreg cell population percentage was similar between WT and Jmjd3 cKO mice (9.7% versus 11.3%; Fig. 1e ). These results suggest that Jmjd3 ablation markedly promotes Th17 and Th2 cell differentiation in the small intestine and colon and decreases Th1 cell differentiation in the small intestine and spleen. However, its effects on lymphatic Th1, Th2, Th17 and Treg cells are relatively small. 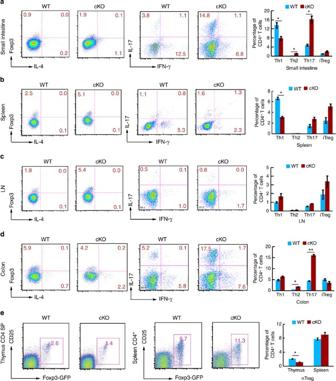Figure 1: Jmjd3 deletion alters CD4+T-cell populations in different organs. Frequency of CD4+T-cell populations isolated from the (a) small intestine, (b) spleen, (c) LN and (d) colon of WT andJmjd3cKO mice. (e) Frequency of thymic and splenic nTreg cell populations (CD25+CD4+GFP+) from WT andJmjd3cKO Foxp3-GFP reporter mice. Mean percentage of the indicated T-cell populations±s.d. shown as histograms (right panel; representative of three independent experiments,n=3 for each group, *P<0.05 determined by Student’st-test). Figure 1: Jmjd3 deletion alters CD4 + T-cell populations in different organs. Frequency of CD4 + T-cell populations isolated from the ( a ) small intestine, ( b ) spleen, ( c ) LN and ( d ) colon of WT and Jmjd3 cKO mice. ( e ) Frequency of thymic and splenic nTreg cell populations (CD25 + CD4 + GFP + ) from WT and Jmjd3 cKO Foxp3-GFP reporter mice. Mean percentage of the indicated T-cell populations±s.d. shown as histograms (right panel; representative of three independent experiments, n =3 for each group, * P <0.05 determined by Student’s t -test). Full size image Jmjd3 alters T-cell differentiation and cytokine expression To determine whether Jmjd3 ablation affects CD4 + T-cell differentiation under different cytokine-polarizing conditions, the percentage of IFN-γ-, IL-4- and IL-17-producing T cells and Foxp3-expressing T cells was analysed in WT and Jmjd3 cKO purified naïve CD4 + T cells cultured under ThN (non-skewing cytokines), Th1 (in the presence of IL-12), Th2 (in the presence of IL-4), Th17 (in the presence of transforming growth factor (TGF-β) and IL-6) and Treg cell (in the presence of TGF-β and IL-2) conditions for 4 days. Jmjd3 ablation reduced the percentage of IFN-γ-producing Th1 cells from 50.1 to 6.2% and increased IL-4-producing Th2 cells from 3.2 to 48.6% under ThN conditions ( Fig. 2a ). Under Th1 conditions, Jmjd3 ablation also reduced the percentage of IFN-γ-producing Th1 cells. The percentage of T cells producing both IFN-γ and IL-4 was slightly higher in Jmjd3 -deficient T cells compared with WT T cells (10.3% versus 6.2%) under ThN conditions and significantly higher under Th1-stimulating cell culture conditions (11.3% versus 2.2%; Fig. 2a ), suggesting that Jmjd3 -deficient T cells are readily differentiated into Th2 cells. Under Th2 conditions, Jmjd3 -deficient T cells slightly increased in their differentiation into IL-4-producing Th2 cells and slightly decreased into IFN-γ-producing Th1 cells or into IFN-γ- and IL-4-producing cells. However, these changes were not statistically significant, suggesting that exogenous cytokines under Th2 conditions may mask the intrinsic difference between WT and Jmjd3 -deficient T cells. Th17 cell differentiation was increased in Jmjd3 -deficient T cells under Th17-stimulating conditions ( Fig. 2b ). In contrast, the inducible Treg cell population was markedly reduced under Treg cell conditions in Jmjd3 -deficient T cells compared with WT T cells (34.3% versus 63.1%; Fig. 2b ). Jmjd3 ablation affects cytokine production of freshly isolated naïve CD4 + T cells stimulated with anti-CD3 and anti-CD28. IFN-γ production was significantly reduced in Jmjd3 -deficient CD4 + T cells at 12, 24 and 48 h ( P <0.01), whereas IL-4 production was markedly increased at 24 and 48 h ( P <0.05 and P <0.01, respectively; Fig. 2c ). To determine whether the increased IL-4 production was due to the early decreased IFN-γ production, we treated cultured T cells with exogenous IFN-γ and measured IL-4 production. Exogenous IFN-γ reduced IL-4 production in both WT and Jmjd3 -deficient T cells; however, the Jmjd3 -deficient T cells still produced higher amounts of IL-4 compared with WT T cells ( Fig. 2d ), suggesting that Jmjd3 -deficient T cells preferentially polarize to Th2. Similarly, exogenous IFN-γ suppressed IL-4-producing Th2 cells in both WT and Jmjd3 -deficient T cells. However, exogenous IFN-γ suppressed IL-4-producing Th2 cells to a greater extent in WT compared with Jmjd3 -deficient T cells ( Fig. 2e ). Taken together, these data indicate that Jmjd3 deficiency results in a Th1 to Th2 shift in the CD4 + T-cell population. 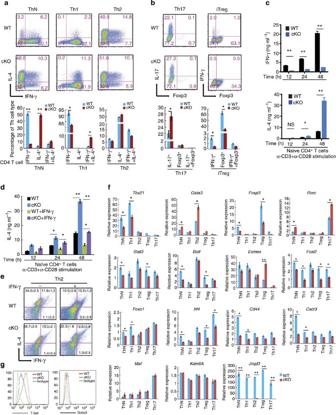Figure 2:Jmjd3ablation alters the differentiation of naïve T cells into Th1, Th2, Th17 and Treg cell lineagesin vitro. (aandb) Frequency of IFN-γ-, IL-4- and IL-17-producing and Foxp3-expressing CD4+T cells after exposure of WT andJmjd3cKO naïve CD4+T cells to ThN, Th1, Th2, Th17 or Treg-inducing conditions. Mean percentage of the indicated T-cell populations±s.d. shown as histograms (bottom panel). (c) IFN-γ (top panel) and IL-4 (bottom panel) production by WT andJmjd3cKO naïve CD4+T cells stimulated with soluble anti-CD3 and anti-CD28 in the presence of T cell-depleted irradiated splenocytes. (d) IL-4 production by WT andJmjd3cKO naïve CD4+T cells under Th2-stimulating cell culture conditions with exogenous addition of IFN-γ. (e) Frequency of Th2 cells after exposure to Th2-stimulating cell culture conditions plus exogenous IFN-γ. (f) Relative gene expression of T-cell differentiation factors from WT andJmjd3cKO naïve CD4+cells cultured under ThN, Th1, Th2, Th17 or Treg-inducing conditions.Xaxis, different cytokine condition;Yaxis, relative expression at mRNA level. (g) Intracellular staining of T-bet and Gata3 in CD4+T cells cultured under ThN conditions (representative of three independent experiments,n=3 for each group, *P<0.05, **P<0.01 determined by Student’st-test). Figure 2: Jmjd3 ablation alters the differentiation of naïve T cells into Th1, Th2, Th17 and Treg cell lineages in vitro . ( a and b ) Frequency of IFN-γ-, IL-4- and IL-17-producing and Foxp3-expressing CD4 + T cells after exposure of WT and Jmjd3 cKO naïve CD4 + T cells to ThN, Th1, Th2, Th17 or Treg-inducing conditions. Mean percentage of the indicated T-cell populations±s.d. shown as histograms (bottom panel). ( c ) IFN-γ (top panel) and IL-4 (bottom panel) production by WT and Jmjd3 cKO naïve CD4 + T cells stimulated with soluble anti-CD3 and anti-CD28 in the presence of T cell-depleted irradiated splenocytes. ( d ) IL-4 production by WT and Jmjd3 cKO naïve CD4 + T cells under Th2-stimulating cell culture conditions with exogenous addition of IFN-γ. ( e ) Frequency of Th2 cells after exposure to Th2-stimulating cell culture conditions plus exogenous IFN-γ. ( f ) Relative gene expression of T-cell differentiation factors from WT and Jmjd3 cKO naïve CD4 + cells cultured under ThN, Th1, Th2, Th17 or Treg-inducing conditions. X axis, different cytokine condition; Y axis, relative expression at mRNA level. ( g ) Intracellular staining of T-bet and Gata3 in CD4 + T cells cultured under ThN conditions (representative of three independent experiments, n =3 for each group, * P <0.05, ** P <0.01 determined by Student’s t -test). Full size image Jmjd3 ablation affects master regulators of T-cell fate We hypothesized that Jmjd3 deletion may alter the expression of key T-cell lineage-specific transcription factors, including T-bet (Th1; encoded by Tbx21 ), Gata3 (Th2), RORγt (Th17; encoded by Rorc ) and Foxp3 (Treg), as well as epigenetic factors and potential target genes. Real-time PCR analysis of T-cell differentiation-related genes was performed on RNA isolated from WT and Jmjd3 -deficient CD4 + T cells cultured under various cytokine-polarizing conditions for 2 days. Tbx21 , Foxo1 , Cd44 and Cxcr3 expression levels were markedly lower under ThN and Th1 cell culture conditions in Jmjd3 -deficient T cells than in WT T cells ( Fig. 2f ). In contrast, Gata3 expression was increased under ThN and Th2 conditions in Jmjd3 -deficient T cells compared with WT T cells ( Fig. 2f ). Foxp3 , Stat3 , Batf , Fosl2 and Irf4 expression levels were lower under ThN and Treg conditions in Jmjd3 -deficient T cells than in WT T cells. Eomes expression was increased under Treg conditions. Fosl2 expression levels were decreased under Th1, Th2 and Th17 conditions. Rorc expression was increased under ThN and Th17 conditions in Jmjd3 -deficient T cells compared with WT T cells. Irf4 expression was lower under ThN, Treg and Th17 conditions in Jmjd3 -deficient T cells than in WT T cells ( Fig. 2f ). In contrast to Tbx21 , Gata3 , Foxp3 , Rorc and Irf4 , little or no difference was observed in Maf and Kdm6A (also known as UTX) expression. Consistent with Tbx21 and Gata3 expression based on real-time PCR results, intracellular staining analysis of T-bet and Gata3 expression also showed a lower level of T-bet and a higher level of Gata3 protein in Jmjd3 -deficient T cells than in WT T cells under ThN culture conditions ( Fig. 2g ). To determine whether chemokines or chemokine receptors, which might affect tissue migration, are changed between WT and Jmjd3 -deficient T cells, CD4 + T cells were isolated from Jmjd3 cKO mice and showed decreased expression of several chemokine receptors, including Ccr2, Ccr4, Ccr8 and Cxcr3 , whereas Ccr9 expression was increased in these cells. However, expression of CD103 and other chemokine receptors was unchanged ( Supplementary Fig. 2 ). Taken together, these results suggest that Jmjd3 ablation inhibits Th1 and Treg differentiation and promotes Th2 and Th17 differentiation by regulating the expression of key transcription factors. Altered expression of chemokine receptors, such as Ccr2, Ccr4, Ccr8, Cxcr3 and Ccr9 , might be responsible for the migration of differentiated T cells to specific sites such as small intestines and colons. Jmjd3 -deficient T cells limit colitis Having established that Jmjd3 ablation alters CD4 + T-cell differentiation in vitro , we next sought to validate these findings in vivo using a Th1-dependent colitis model. Intraperitoneal (i.p.) adoptive transfer of freshly isolated and purified naïve WT CD4 + T cells into lymphopenic Rag2 −/− γc −/− mice caused spontaneous T-cell activation and inflammatory colitis, leading to body weight loss ( Fig. 3a ). In contrast, Rag2 −/− γc −/− mice receiving naïve CD4 + T cells from Jmjd3 cKO mice developed a milder colitis, with a body weight loss less than that of mice receiving WT T cells ( Fig. 3a ). FACS analysis of splenic and intestinal CD4 + T cells revealed a marked increase in IL-4-producing Th2 cells and a decrease in IFN-γ-producing Th1 cells in Rag2 −/− γc −/− mice receiving Jmjd3 -deficient T cells compared with those receiving WT CD4 + T cells ( Fig. 3b ). Consistently, IFN-γ-producing Th1 cells were decreased in Rag2 −/− γc −/− mice receiving intravenous Jmjd3 cKO naïve CD4 + T cells compared with those receiving WT CD4 + T cells ( Fig. 3c ). To further determine the role of Jmjd3 -deficient Th1 cells in the colitis models with or without Treg cells from WT and Jmjd3 -deficient mice, we isolated and transferred WT or Jmjd3 -deficient CD4 + T cells into lymphopenic Rag2 −/− γc −/− mice, and measured percent initial body weight change. Consistent with our findings in Fig. 3a , Jmjd3 -deficient T cells limited colitis in Rag2 −/− γc −/− mice ( Fig. 3d ). To determine whether Jmjd3 deficiency affects Treg cell suppressive function in the Th1-mediated colitis model, we isolated and transferred WT and Jmjd3 -deficient Treg cells together with naïve WT CD4 + T cells into lymphopenic Rag2 −/− γc −/− mice. Co-transfer of both naïve CD4 + T cells and Treg cells suppressed weight loss and decreased colitis score at 40 days post-cell transfer regardless of whether the Treg cells were derived from WT or Jmjd3 -deficient mice ( Fig. 3d–f ). Jmjd3 ablation inhibits Th1 differentiation and promotes Th2 differentiation in an in vivo colitis model, but does not affect the suppressive function of Treg cells. 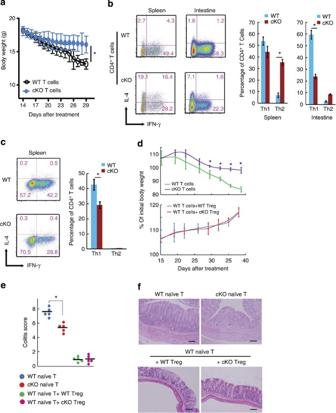Figure 3:Jmjd3ablation promotes Th2 differentiation and suppresses Th1 differentiationin vivo. (a) Naïve CD4+T cells (CD4+CD25−CD62L+CD44low) from WT andJmjd3 cKO mice were FACS-purified and i.p. injected into irradiatedRag2−/−γc−/−mice (2 × 106cells per mouse). Body weight loss was monitored daily, indicating colitis progression (data are expressed as mean±s.d. from three independent experiments,n=5 mice in each group, *P<0.05). (b) Percentages of splenic and colonic IL-4- and IFN-γ-producing CD4+T cells from mice with colitis, one month following adoptive transfer of WT andJmjd3 cKO naïve CD4+T cells. Mean percentage of indicated T-cell populations±s.d. shown as histograms (right panel;n=3 mice per group, *P<0.05). (c) WT andJmjd3cKO naïve CD4+T cells (2 × 106) were i.v. injected into irradiatedRag2−/−γc−/−mice. Ten days later, frequency of IL-4- and IFN-γ-producing T cells from isolated splenocytes. Mean percentage of the indicated cell populations±s.d. as shown by histograms (right panel; representative results from at least three independent experiments,n=3 per group, *P<0.05). (d) Naïve CD4+T cells and nTreg cells (CD4+CD25+) from WT andJmjd3 cKO mice were FACS-purified and i.p. injected intoRag2−/−γc−/−mice (1 × 106T cells+0.2 × 106nTreg cells per mouse). Body weight loss was monitored daily for colitis progression and reported as the mean±s.d. from three independent experiments (n=5 mice in each group, *P<0.05). (e) Colitis score for individualRag2−/−γc−/−mice (points) receiving indicated T cells and Treg cells (n=5 mice in each group, *P<0.05 determined by Student’st-test). (f) H&E staining of colon fromRag2−/−γc−/−mice receiving indicated T cells. Scale bar, 200 μm. Figure 3: Jmjd3 ablation promotes Th2 differentiation and suppresses Th1 differentiation in vivo . ( a ) Naïve CD4 + T cells (CD4 + CD25 − CD62L + CD44 low ) from WT and Jmjd 3 cKO mice were FACS-purified and i.p. injected into irradiated Rag2 −/− γc −/− mice (2 × 10 6 cells per mouse). Body weight loss was monitored daily, indicating colitis progression (data are expressed as mean±s.d. from three independent experiments, n =5 mice in each group, * P <0.05). ( b ) Percentages of splenic and colonic IL-4- and IFN-γ-producing CD4 + T cells from mice with colitis, one month following adoptive transfer of WT and Jmjd 3 cKO naïve CD4 + T cells. Mean percentage of indicated T-cell populations±s.d. shown as histograms (right panel; n =3 mice per group, * P <0.05). ( c ) WT and Jmjd3 cKO naïve CD4 + T cells (2 × 10 6 ) were i.v. injected into irradiated Rag2 −/− γc −/− mice. Ten days later, frequency of IL-4- and IFN-γ-producing T cells from isolated splenocytes. Mean percentage of the indicated cell populations±s.d. as shown by histograms (right panel; representative results from at least three independent experiments, n =3 per group, * P <0.05). ( d ) Naïve CD4 + T cells and nTreg cells (CD4 + CD25 + ) from WT and Jmjd 3 cKO mice were FACS-purified and i.p. injected into Rag2 −/− γc −/− mice (1 × 10 6 T cells+0.2 × 10 6 nTreg cells per mouse). Body weight loss was monitored daily for colitis progression and reported as the mean±s.d. from three independent experiments ( n =5 mice in each group, * P <0.05). ( e ) Colitis score for individual Rag2 −/− γc −/− mice (points) receiving indicated T cells and Treg cells ( n =5 mice in each group, * P <0.05 determined by Student’s t -test). ( f ) H&E staining of colon from Rag2 −/− γc −/− mice receiving indicated T cells. Scale bar, 200 μm. Full size image Jmjd3 ablation reduces T-cell plasticity CD4 + T cells show remarkable plasticity and can differentiate into multiple T-cell lineages depending on the local cytokine milieu [2] . To determine the effects of Jmjd3 deficiency on T-cell plasticity, CD4 + Th1 cells were generated from naïve WT and Jmjd3 -deficient T cells under Th1 conditions with subsequent exposure to Th2, Th17 or Treg-inducing conditions. Compared with Jmjd3 -deficient Th1 cells, a lower percentage of WT Th1 cells were converted into IL-4-producing Th2 T cells, including IL-4-only-producing (2.6% versus 10.7%) and IL-4/IFN-γ double-producing (3.6% versus 10.0%) T cells ( Fig. 4a ). Similarly, a lower percentage of WT Th1 cells converted into IL-17-producing Th17 T cells, but a similar percentage of WT Th1 cells converted into Treg cells, compared with Jmjd3 -deficient cells ( Fig. 4a ). 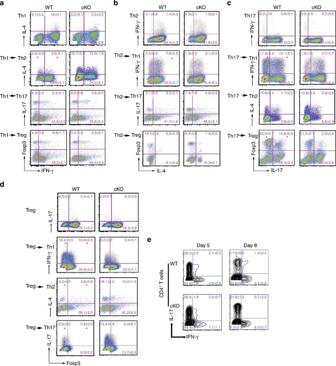Figure 4:Jmjd3ablation increases Th2, Th17 and Treg cell stabilityin vitro. (a) WT andJmjd3 cKO naïve CD4+T cells were differentiated under Th1-inducing conditions for 3 days, and then exposed to Th2, Th17 or Treg-inducing cell culture conditions for 3 days. Frequency of IFN-γ-, IL-4-, IL-17- and Foxp3-producing CD4+T cells. (b) WT andJmjd3 cKO naïve CD4+T cells were differentiated under Th2 conditions for 3 days, and then exposed to Th1, Th17 or Treg-inducing cell culture conditions for 3 days. Frequency of IFN-γ-, IL-4-, IL-17- and Foxp3-producing CD4+T cells. (c) WT andJmjd3 cKO naïve CD4+T cells were differentiated under Th17 conditions for 3 days, and then exposed to Th1, Th2 and Treg-inducing cell culture conditions for 3 days. Frequency of IFN-γ-, IL-4-, IL-17- and Foxp3-producing CD4+T cells. (d) Naïve CD4+T cells derived from WT andJmjd3cKOFoxp3-GFPreporter mice were differentiated under Treg conditions for 4 days. GFP+cells were sorted and cultured under Th1, Th2 or Th17-inducing conditions for 2 days. Frequency of Foxp3-GFP+, IL-4-, IL-17- and IFN-γ-producing CD4+T cells. (e) WT andJmjd3cKO mice were i.v. injected with anti-CD3 to inducein vivoTh17 differentiation. Frequency of IL-17- and IFN-γ-producing CD4+T cells from lymphocytes isolated from the small intestine, day 5 and day 8 after injection (representative of three independent experiments, *P<0.05 determined by Student’st-test). Figure 4: Jmjd3 ablation increases Th2, Th17 and Treg cell stability in vitro . (a ) WT and Jmjd 3 cKO naïve CD4 + T cells were differentiated under Th1-inducing conditions for 3 days, and then exposed to Th2, Th17 or Treg-inducing cell culture conditions for 3 days. Frequency of IFN-γ-, IL-4-, IL-17- and Foxp3-producing CD4 + T cells. ( b ) WT and Jmjd 3 cKO naïve CD4 + T cells were differentiated under Th2 conditions for 3 days, and then exposed to Th1, Th17 or Treg-inducing cell culture conditions for 3 days. Frequency of IFN-γ-, IL-4-, IL-17- and Foxp3-producing CD4 + T cells. ( c ) WT and Jmjd 3 cKO naïve CD4 + T cells were differentiated under Th17 conditions for 3 days, and then exposed to Th1, Th2 and Treg-inducing cell culture conditions for 3 days. Frequency of IFN-γ-, IL-4-, IL-17- and Foxp3-producing CD4 + T cells. ( d ) Naïve CD4 + T cells derived from WT and Jmjd3 cKO Foxp3-GFP reporter mice were differentiated under Treg conditions for 4 days. GFP + cells were sorted and cultured under Th1, Th2 or Th17-inducing conditions for 2 days. Frequency of Foxp3-GFP + , IL-4-, IL-17- and IFN-γ-producing CD4 + T cells. ( e ) WT and Jmjd3 cKO mice were i.v. injected with anti-CD3 to induce in vivo Th17 differentiation. Frequency of IL-17- and IFN-γ-producing CD4 + T cells from lymphocytes isolated from the small intestine, day 5 and day 8 after injection (representative of three independent experiments, * P <0.05 determined by Student’s t -test). Full size image Next, we investigated Jmjd3 -deficient Th2 cell plasticity. CD4 + Th2 cells were generated from naïve WT and Jmjd3 -deficient T cells under Th2 conditions with subsequent exposure to Th1, Th17 or Treg-inducing conditions. Th2-conditioned WT cells more readily converted to IFN-γ-producing Th1 cells and Foxp3-expressing Treg cells than Th2-conditioned Jmjd3 -deficient T cells. A lower percentage of WT Th2 cells converted to IL-17-producing Th17 cells, compared with Jmjd3 -deficient cells ( Fig. 4b ). Differentiated Jmjd3 -deficient Th17 cells were exposed to Th1-, Th2- or Treg-inducing conditions. Compared with Jmjd3 -deficient Th17 cells, a greater percentage of WT Th17 cells converted to IFN-γ-producing Th1 T cells, including IFN-γ-only-producing (11.8% versus 1.9%) and IFN-γ/IL-17 double-producing (12.1% versus 5.7%) T cells ( Fig. 4c ). A higher percentage of WT Th17 cells were also converted to Treg cells, and a lower percentage converted to double-positive IL-4/IL-17 cells compared with Jmjd3 -deficient cells ( Fig. 4c ). We also examined the plasticity of Treg cells differentiated from WT and Jmjd3 -deficient mice. Naïve CD4 + T cells isolated from WT and Jmjd3 cKO mice were differentiated under Treg conditions for 4 days, and then exposed to Th1-, Th2- or Th17-inducing conditions for 2 days. Treg cell conversion into IFN-γ-producing cells and IFN-γ/Foxp3-producing Th1 cells decreased from 12.4 to 3.2% and 10.8 to 2.4%, respectively, in Jmjd3 cKO T cells compared with WT T cells. Treg cell conversion into IL-17-producing cells and IL-17/Foxp3-producing cells increased from 2.6 to 10.4% and 0.5 to 2.4%, respectively, in Jmjd3 cKO T cells compared with WT T cells. ( Fig. 4d ). A slightly lower percentage of WT Treg cells, compared with Jmjd3 cKO cells, were converted to Th2 cells ( Fig. 4d ). Furthermore, using an anti-CD3 antibody-induced mouse model of tolerance [42] , we showed a dramatic increase in intestinal Th17 cells in Jmjd3 cKO T cells at day 8 after in vivo Th17 differentiation compared with WT T cells ( Fig. 4e ). Taken together, our results suggest that Jmjd3 is required for Th1 differentiation, and its ablation reduces the plasticity of Th2, Th17 and Treg cell conversion into Th1 cells. Decreased T-bet, CD44 and CXCR3 in Jmjd3 -cKO T cells As T-bet is a critical transcription factor for Th1 cell differentiation [43] , we next investigated Jmjd3 regulation of T-bet and its target genes. CD44 is expressed at an early stage in T-cell development in the thymus, and is regulated by Jmjd3 (ref. 42 ). Indeed, we found that CD44 expression was significantly decreased in Jmjd3 -deficient ThN and Th1 cells, single-positive (SP) CD4 + thymocytes and splenocytes ( Fig. 2f , Supplementary Fig. 2 ). We further analysed CD44 low (CD44 − ) and CD44 high (CD44 + ) CD4 + SP thymic T-cell populations and determined T-bet expression by FACS analysis. T-bet protein was reduced in the Jmjd3 -deficient CD44 high T-cell population compared with the WT CD44 high T-cell population, whereas little or no T-bet was detected in the WT or Jmjd3 -deficient CD44 low T-cell population ( Fig. 5a ). Furthermore, we found downregulated CD44 and CXCR3 (T-bet target genes) expression, or fewer numbers of cells expressing CD44, in Jmjd3 -deficient T cells compared with WT T cells ( Fig. 5b,c ). To validate our findings in vivo , CXCR3 and CD44 expression levels were determined in splenocytes isolated from Rag2 −/− γc −/− mice injected with WT or Jmjd3 cKO naïve CD4 + T cells. Percentage of T cells, expressing both CXCR3 and CD44, was downregulated in Jmjd3 -deficient T cells compared with WT T cells ( Fig. 5d ). These findings suggest that Jmjd3 deletion reduces the expression of T-bet, CXCR3 and CD44 in CD4 + T cells, or Jmjd3 -deficient T cells contain fewer cells expressing T-bet, CXCR3 and CD44. 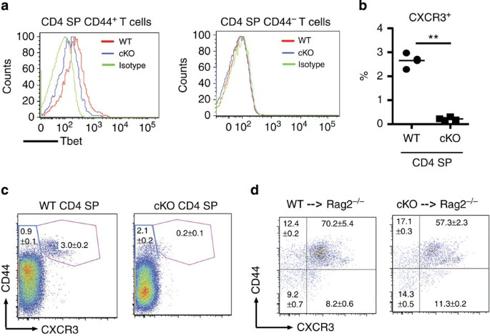Figure 5: Jmjd3 regulates CD44 and CXCR3 in CD4+T cells. (a) T-bet protein expression in WT andJmjd3cKO CD44+and CD44−CD4 SP thymocytes. (b) Percentage of CXCR3+cells in CD4+SP T cells from WT andJmjd3cKO mice (data expressed as mean+s.d. of three independent experiments, *P<0.05, **P<0.01). (c) Frequency of CD44 and CXCR3 in WT andJmjd3cKO CD4+SP thymocytes. (d) Naïve CD4+T cells (2 × 106) derived from WT andJmjd3cKO mice were i.v. injected into irradiatedRag2−/−γc−/−mice (n=3 for each group). Ten days later, frequency of CD44+CXCR3+-expressing T cells isolated from splenocytes (representative of three independent experiments, *P<0.05, **P<0.01 determined by Student’st-test). Figure 5: Jmjd3 regulates CD44 and CXCR3 in CD4 + T cells. ( a ) T-bet protein expression in WT and Jmjd3 cKO CD44 + and CD44 − CD4 SP thymocytes. ( b ) Percentage of CXCR3 + cells in CD4 + SP T cells from WT and Jmjd3 cKO mice (data expressed as mean+s.d. of three independent experiments, * P <0.05, ** P <0.01). ( c ) Frequency of CD44 and CXCR3 in WT and Jmjd3 cKO CD4 + SP thymocytes. ( d ) Naïve CD4 + T cells (2 × 10 6 ) derived from WT and Jmjd3 cKO mice were i.v. injected into irradiated Rag2 −/− γc −/− mice ( n =3 for each group). Ten days later, frequency of CD44 + CXCR3 + -expressing T cells isolated from splenocytes (representative of three independent experiments, * P <0.05, ** P <0.01 determined by Student’s t -test). Full size image Jmjd3 alters target gene methylation of H3K27 and H3K4 To determine the mechanisms by which Jmjd3 regulates target gene expression, we tested whether Jmjd3 ablation affects global histone methylation in T cells. H3K27me2 and H3K27me3, but not H3K27me1, levels were increased in Jmjd3 -deficient thymic CD4 + SP T cells compared with WT, whereas appreciable changes in H3K4 methylation were not observed ( Fig. 6a , Supplementary Fig. 3a , and Supplementary Table 1 ). This suggests that Jmjd3 deletion specifically increases H3K27 dimethylation and trimethylation in CD4 + T cells. ChIP-Seq analysis on WT and Jmjd3 -deficient CD4 + T cells revealed that among the 35,000 RefSeq genes, 2,754 genes had increased H3K27me3 levels at approximately 2 kilobases around the transcription start site (TSS) in Jmjd3 -deficient CD4 + T cells compared with WT controls. H3K27me3 levels were decreased in 811 genes ( Fig. 6b and Supplementary Table 1 ). H3K4me3 levels were increased in 404 genes and decreased in 114 genes in Jmjd3 -deficient CD4 + T cells compared with WT ( Fig. 6b and Supplementary Table 1 ). Analysis of average H3K27me3 levels of the differentially methylated genes revealed that total H3K27me3 methylation levels were increased in both promoter regions and gene bodies in Jmjd3 -deficient CD4 + T cells compared with WT cells ( Fig. 6c ). H3K4me3 is generally correlated with active transcription, whereas H3K27me3 is associated with gene repression. Chromatin regions containing high levels of both H3K4me3 and H3K27me3 are known as ‘bivalent domains’, which are silenced and postulated to be ‘poised’ for activation [44] , [45] . T cell-related genes were classified into three groups according to H3K27me3 and H3K4me3 status, and significant differences were found between WT and Jmjd3 -deficient CD4 + T cells. Group I genes, including Cd44 , Ccnd2 , Ifng , Irf4 , Ccr2 and Fosl2 , in Jmjd3 -deficient CD4 + T cells, harboured bivalent domains with increased H3K27me3 and decreased H3K4me3 levels ( Fig. 6d and Supplementary Fig. 4a ), which paralleled decreased gene expression. Group II genes, including Foxp3 , Stat3 , Tgfß1 , Cxcr3 , Cxcr6 , Ccr8 and Ccr4 , had decreased H3K4me3 and unchanged H3K27me3 levels in Jmjd3 -deficient CD4 + T cells, which paralleled their decreased gene expression ( Fig. 6d and Supplementary Fig. 4b ). Conversely, in group III genes, Tbx21, Gata3 , Rorc, Smad3 , Maf and several chemokine receptors, both H3K27me3 and H3K4me3 levels were not dramatically changed ( Fig. 6d and Supplementary Fig. 4c ). These histone methylation changes were further validated using chromatin immunoprecipitation (ChIP)-quantitative PCR (qPCR; Fig. 6e ). We found only a few genes that had histone methylation changes at distal regions ( Supplementary Fig. 5 ). These results suggest that Jmjd3 regulates target gene expression primarily through alterations in the histone methylation status of H3K27 and/or H3K4 in the promoter and gene body regions. 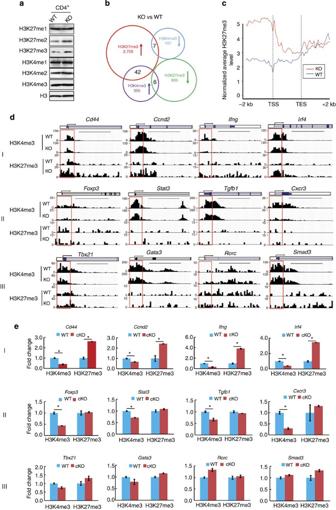Figure 6: Jmjd3 regulates target gene expression by altering H3K4me3 and H3K27me3 levels. (a) Western blot of global H3K4me1/me2/me3 and H3K27me1/me2/me3 levels in thymic CD4+SP T cells. (b) H3K4me3 and H3K27me3 in WT andJmjd3cKO CD4 SP T cells were analysed by genome-wide ChIP-Seq. Venn diagram showing the numbers of genes with H3K27me3 and H3K4me3 modifications inJmjd3cKO cells compared with WT cells. (c) Average H3K27me3 profiles in WT and cKO samples at differentially methylated genes. TSS, transcription start site; TES, transcription end site. (d) T cell-related genes were classified into three groups based on H3K4me3 and H3K27me3 modifications in WT andJmjd3cKO CD4 SP thymocytes: group I, increased H3K27 and decreased H3K4; group II, unchanged H3K27 and decreased H3K4; and group III, unchanged H3K27 and H3K4. Red frames indicate the 2 kb region around the TSS. Scale bars represent 5 kb region. (e) Validation of methylation changes in WT and cKO CD4 SP thymocytes by ChIP-qPCR (*P<0.05 determined by Student’st-test). Figure 6: Jmjd3 regulates target gene expression by altering H3K4me3 and H3K27me3 levels. ( a ) Western blot of global H3K4me1/me2/me3 and H3K27me1/me2/me3 levels in thymic CD4 + SP T cells. ( b ) H3K4me3 and H3K27me3 in WT and Jmjd3 cKO CD4 SP T cells were analysed by genome-wide ChIP-Seq. Venn diagram showing the numbers of genes with H3K27me3 and H3K4me3 modifications in Jmjd3 cKO cells compared with WT cells. ( c ) Average H3K27me3 profiles in WT and cKO samples at differentially methylated genes. TSS, transcription start site; TES, transcription end site. ( d ) T cell-related genes were classified into three groups based on H3K4me3 and H3K27me3 modifications in WT and Jmjd3 cKO CD4 SP thymocytes: group I, increased H3K27 and decreased H3K4; group II, unchanged H3K27 and decreased H3K4; and group III, unchanged H3K27 and H3K4. Red frames indicate the 2 kb region around the TSS. Scale bars represent 5 kb region. ( e ) Validation of methylation changes in WT and cKO CD4 SP thymocytes by ChIP-qPCR (* P <0.05 determined by Student’s t -test). Full size image Jmjd3 interacts with transcription and epigenetic factors We next determined whether Jmjd3 recruitment to specific gene promoters was mediated through interactions with transcription and epigenetic factors involved in T-cell differentiation. Co-immunoprecipitation analyses revealed that Jmjd3 interacts with T-bet, but not Gata3, Foxp3 or RoRγt, in 293T cells ( Fig. 7a and Supplementary Fig. 3b ). Because H3K4 methylation levels were altered at many gene loci in Jmjd3 -deficient T cells, we determined its interaction with key components of the H3K4 methyltransferase complex (Ash2L, RbBP5 and Wdr5). We found that Jmjd3 interacted with Ash2L, but not with RbBP5 or Wdr5, in 293T cells ( Fig. 7b and Supplementary Fig. 3c ). Co-immunoprecipitation in 293T cells, co-transfected with T-bet and FLAG -tagged Ash2L , RbBP5 and Wdr5 plasmids, revealed that T-bet physically interacted with RbBP5 ( Fig. 7c and Supplementary Fig. 3d ). The endogenous interaction of Jmjd3 with Ash2L and T-bet was observed in WT but not in Jmjd3 cKO T cells ( Fig. 7d and Supplementary Fig. 3e ). Although T-bet interacts with Jmjd3 and RbBP5, a core protein of the H3K4 methyltransferase complex [39] , it is unclear whether Jmjd3 is required for T-bet–RbBP5 interaction. Immunoprecipitation and immunoblot analysis revealed that T-bet interacted with RbBP5 in the presence of Jmjd3, but failed to interact in Jmjd3 -deficient T cells ( Fig. 7e and Supplementary Fig. 3f ). To determine the functional relevance, we performed ChIP-qPCR) analysis of Cxcr3 and Ifng promoter regions in WT and Jmjd3 cKO Th1 cells and CD4 + SP thymocytes. Consistent with our previous observations, Jmjd3 -deficient T cells disrupted the endogenous T-bet–RbBP5 interaction and markedly reduced T-bet binding to the promoter regions of Cxcr3 , Ifng and Cd44 genes ( Fig. 7f and Supplementary Fig. 6a ). These results suggest that Jmjd3 is required for T-bet and Ash2L to form a stable complex capable of binding to specific target gene promoters. Jmjd3 deficiency might destabilize this complex formation and reduce T-bet binding to Cxcr , Ifng and Cd44 promoters, leading Cxcr3 , Ifng and Cd44 gene expression downregulation. 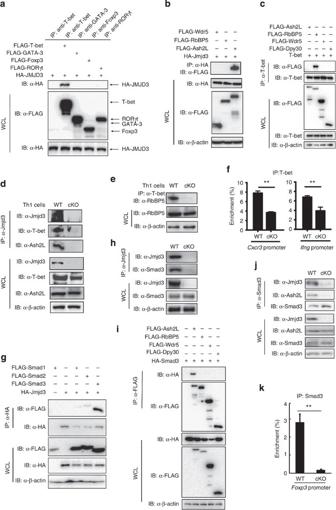Figure 7: Jmjd3 regulates Th1 and Th2 differentiation by facilitating the T-bet–RbBP5 and Smad3–Ash2L interaction. (a) 293T cells were co-transfected with HA-Jmjd3 and FLAG-tagged T-bet, GATA-3, Foxp3 and RORγT plasmids. Whole-cell lysates (WCLs) were immunoprecipitated with anti-T-bet, anti-GATA-3, anti-Foxp3 and anti-RORγT antibodies and immunoblotted with anti-FLAG antibody. (b) 293T cells were co-transfected with HA-Jmjd3- and FLAG-tagged Wdr5, Ash2L or RbBP5. WCL were immunoprecipitated with anti-HA beads and immunoblotted with anti-FLAG antibody. (c) 293T cells were co-transfected with T-bet and FLAG-tagged Wdr5, Ash2L, Dpy30 or RbBP5. WCL were immunoprecipitated with anti-T-bet antibody and protein (A+G) beads, and immunoblotted with anti-FLAG antibody. (d) Cell lysates were obtained from WT andJmjd3cKO Th1 cells and immunoprecipitated with anti-Jmjd3 antibody and protein (A+G) beads. The immunoprecipitated product was immunoblotted with anti-Jmjd3, anti-T-bet and anti-Ash2L antibodies. (e) WCL were obtained from WT andJmjd3cKO Th1 cells and immunoprecipitated with anti-T-bet antibody and protein (A+G) beads. The immunoprecipitated product was immunoblotted with anti-RbBP5 antibody. (f) ChIP-qPCR analysis of T-bet binding to the promoter regions ofCxcr3andIfnggenes in WT andJmjd3cKO Th1 cells. (g) WCL obtained from 293T cells co-transfected with HA-Jmjd3 and FLAG-Smad1, FLAG-Smad2 or FLAG-Smad3 plasmids were immunoprecipitated with anti-HA beads. The immunoprecipitated product was immunoblotted with anti-FLAG and anti-HA antibodies. (h) WCL and protein isolates from WT andJmjd3cKO CD4+T cells derived from thymus. (i) 293T cells were co-transfected with HA-tagged Smad3 and FLAG-tagged Wdr5, Ash2L, Dpy30 or RbBP5. WCLs were immunoprecipitated with anti-FLAG beads and immunoblotted with anti-HA antibody. (j) Cell lysates were obtained from WT andJmjd3cKO Treg cells and immunoprecipitated with anti-Smad3 antibody. The immunoprecipitated product was immunoblotted with anti-Jmjd3, anti-Smad3 and anti-Ash2L antibodies. (k) ChIP-qPCR analysis of Smad3 binding to the promoter regions ofFoxp3gene in WT andJmjd3cKO Treg cells. Figure 7: Jmjd3 regulates Th1 and Th2 differentiation by facilitating the T-bet–RbBP5 and Smad3–Ash2L interaction. ( a ) 293T cells were co-transfected with HA-Jmjd3 and FLAG-tagged T-bet, GATA-3, Foxp3 and RORγT plasmids. Whole-cell lysates (WCLs) were immunoprecipitated with anti-T-bet, anti-GATA-3, anti-Foxp3 and anti-RORγT antibodies and immunoblotted with anti-FLAG antibody. ( b ) 293T cells were co-transfected with HA-Jmjd3- and FLAG-tagged Wdr5, Ash2L or RbBP5. WCL were immunoprecipitated with anti-HA beads and immunoblotted with anti-FLAG antibody. ( c ) 293T cells were co-transfected with T-bet and FLAG-tagged Wdr5, Ash2L, Dpy30 or RbBP5. WCL were immunoprecipitated with anti-T-bet antibody and protein (A+G) beads, and immunoblotted with anti-FLAG antibody. ( d ) Cell lysates were obtained from WT and Jmjd3 cKO Th1 cells and immunoprecipitated with anti-Jmjd3 antibody and protein (A+G) beads. The immunoprecipitated product was immunoblotted with anti-Jmjd3, anti-T-bet and anti-Ash2L antibodies. ( e ) WCL were obtained from WT and Jmjd3 cKO Th1 cells and immunoprecipitated with anti-T-bet antibody and protein (A+G) beads. The immunoprecipitated product was immunoblotted with anti-RbBP5 antibody. ( f ) ChIP-qPCR analysis of T-bet binding to the promoter regions of Cxcr3 and Ifng genes in WT and Jmjd3 cKO Th1 cells. ( g ) WCL obtained from 293T cells co-transfected with HA-Jmjd3 and FLAG-Smad1, FLAG-Smad2 or FLAG-Smad3 plasmids were immunoprecipitated with anti-HA beads. The immunoprecipitated product was immunoblotted with anti-FLAG and anti-HA antibodies. ( h ) WCL and protein isolates from WT and Jmjd3 cKO CD4 + T cells derived from thymus. ( i ) 293T cells were co-transfected with HA-tagged Smad3 and FLAG-tagged Wdr5, Ash2L, Dpy30 or RbBP5. WCLs were immunoprecipitated with anti-FLAG beads and immunoblotted with anti-HA antibody. ( j ) Cell lysates were obtained from WT and Jmjd3 cKO Treg cells and immunoprecipitated with anti-Smad3 antibody. The immunoprecipitated product was immunoblotted with anti-Jmjd3, anti-Smad3 and anti-Ash2L antibodies. ( k ) ChIP-qPCR analysis of Smad3 binding to the promoter regions of Foxp3 gene in WT and Jmjd3 cKO Treg cells. Full size image Smad3 has been reported to enhance Treg cell differentiation and inhibit Th17 cell differentiation [46] . Immunoprecipitation analysis revealed that Jmjd3 strongly and specifically interacts with Smad3, but not Smad1 or Smad2, in 293T cells ( Fig. 7g and Supplementary Fig. 3g ). This interaction was also observed in WT, but not in cKO CD4 + T cells derived from thymus ( Fig. 7h and Supplementary Fig. 3h,6b ). To identify a potential link between Jmjd3 deficiency and H3K4 methylation in the Foxp3 promoter region, we found specific interactions between Smad3 and Ash2L of the H3K4 methyltransferase complex ( Fig. 7i and Supplementary Fig. 3i ), which was further confirmed in Treg cells ( Supplementary Fig. 6c ). Immunoprecipitation analysis revealed that Smad3 interacted with Ash2L in the presence of Jmjd3, but failed to interact in Jmjd3 -deficient Treg cells, suggesting that Jmjd3 is required for Smad3–Ash2L interaction ( Fig. 7j and Supplementary Fig. 3j ). These results suggest that Jmjd3 specifically controls Smad3 target gene expression by interacting with epigenetic factors such as Ash2L. To further test this notion, we performed ChIP-qPCR analysis of Foxp3 promoter in WT and Jmjd3 cKO Treg cells. Consistent with our previous observations, Jmjd3 -deficiency dramatically reduced Smad3 binding to Foxp3 promoter regions ( Fig. 7k ). Taken together, Jmjd3 regulates Foxp3 expression by stabilizing the Smad3–Ash2L–Jmjd3 complex. To further validate the functional significance of the physical interactions between Jmjd3 and the transcription factors, we ectopically expressed Jmjd3 in CD4 + T cells under different cytokine conditions. Ectopic expression of Jmjd3 rescued transcription factor and target gene expression ( Fig. 8a , Supplementary Fig. 7 ). ChIP-qPCR analysis revealed that Jmjd3 expression also rescued the binding of the T-bet to Cxcr3 , Ifng and Cd44 promoter regions, and restored the binding of Smad3 to the Foxp3 promoter ( Fig. 8b,c ). Taken together, our results indicate that Jmjd3 regulates T-cell differentiation by interacting with specific transcription and epigenetic factors. 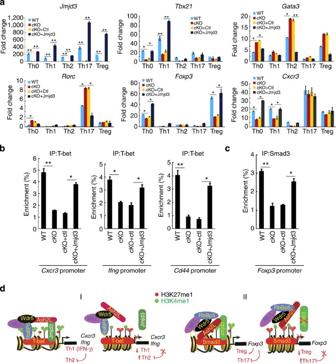Figure 8: Jmjd3 functionally regulates gene expression and DNA binding. (a) Ectopically expressed Jmjd3 rescues the gene expression in Jmjd3-deficient T cells. (b,c) Ectopically expressed Jmjd3 enhances the binding of the transcription factors, T-bet and Smad3, to their target genes (*P<0.05, **P<0.01, determined by Student's t-test). (d) Schematic diagram illustrating the proposed mechanistic role of Jmjd3 in the regulation of CD4+T-cell differentiation. Jmjd3 interacts with T-bet RbBP5 and Ash2L to form a stable complex with transcription factors capable of binding to target gene promoters, thus allowing Jmjd3 to alter H3K27 methylation and Ash2L/RbBP5 to alter H3K4 levels to control target gene expression. Jmjd3 upregulates the expression of Th1 and Treg cell differentiation factors, includingFoxp3,Ifng,Cd44andCxcr3, and downregulates the expression of the Th2 cell differentiation factorsRorcandGata3.These changes in gene expression lead to the promotion of Th1 and Treg cell differentiation and the inhibition of Th2 and Th17 cell differentiation. Figure 8: Jmjd3 functionally regulates gene expression and DNA binding. ( a ) Ectopically expressed Jmjd3 rescues the gene expression in Jmjd3-deficient T cells. ( b , c ) Ectopically expressed Jmjd3 enhances the binding of the transcription factors, T-bet and Smad3, to their target genes (* P <0.05, ** P <0.01, determined by Student's t-test). ( d ) Schematic diagram illustrating the proposed mechanistic role of Jmjd3 in the regulation of CD4 + T-cell differentiation. Jmjd3 interacts with T-bet RbBP5 and Ash2L to form a stable complex with transcription factors capable of binding to target gene promoters, thus allowing Jmjd3 to alter H3K27 methylation and Ash2L/RbBP5 to alter H3K4 levels to control target gene expression. Jmjd3 upregulates the expression of Th1 and Treg cell differentiation factors, including Foxp3 , Ifng , Cd44 and Cxcr3 , and downregulates the expression of the Th2 cell differentiation factors Rorc and Gata3. These changes in gene expression lead to the promotion of Th1 and Treg cell differentiation and the inhibition of Th2 and Th17 cell differentiation. Full size image CD4 + T-cell subsets (Th1, Th2, Th17 and Treg cells) play an important role in cancer immunity and infectious and autoimmune diseases [2] , [16] . Understanding the mechanisms that regulate and control T-cell differentiation will lead to the development of innovative and effective strategies. It is known that the differentiation of naïve CD4 + T cells into the various T-cell subsets is tightly regulated by various signalling molecules; however, the epigenetic regulation of T-cell differentiation remains poorly understood. Recent studies have suggested that epigenetic factors play an important role in CD4 + T-cell differentiation [47] , [48] , [49] . Mixed-lineage leukaemia-mediated H3K4 trimethylation has been implicated in the selective maintenance of memory Th2 cells to produce Th2 cytokines [49] , whereas the histone-lysine N -methyltransferase, Suv39h1, plays a critical role in maintaining the silencing of Th1 loci and modulating Th2 lineage stability and plasticity [47] . Our study provides evidence of the critical role of histone demethylase Jmjd3 in the epigenetic regulation of CD4 + T-cell differentiation. T cell-specific Jmjd3 ablation inhibited Th1 and Treg cell differentiation and promoted Th2 and Th17 cell differentiation by regulating the expression of key T-cell differentiation and transcription factors. In particular, the Th17 cell population is markedly increased in the small intestine and colon, but not in the LN or spleen. We show that Jmjd3 regulates CD4 + T-cell differentiation by controlling the methylation status of H3K27 and/or H3K4 in the promoter and body regions of target genes. Importantly, Jmjd3 is recruited to target gene loci through interactions with the transcription factors, T-bet and Smad3, and the epigenetic protein, Ash2L. However, it is not clear why Jmjd3 ablation has differential effects on different T-cell subsets in different tissues. Thus, further investigation is required to address this issue. Jmjd3 has been shown to regulate gene expression in a demethylase activity-independent [35] , [40] and -dependent manner [37] , [38] , [50] . To our knowledge, our study is the first to provide in vivo evidence of the essential role of Jmjd3 in Th1 and Treg cell differentiation through the demethylase-dependent regulation of Tbx21 (T-bet), Gata3 and Foxp3 expression. ChIP-Seq analysis showed a slight decrease in H3K4me3 in the promoter and gene body of Tbx21 , Gata3 and Foxp3 , whereas H3K4me3 and H3K27me3 levels in the promoter or gene body of Rorc were unchanged even though its expression was increased in Treg and Th17 cells. Tbx21 target gene expression decreased in Jmjd3 -deficient T cells, whereas Jmjd3 and T-bet binding to the Tbx21 target gene promoter were abolished. Our findings indicate that Jmjd3 regulates Th1 differentiation through two mechanisms: (i) direct regulation of Tbx21 expression in a Jmjd3 demethylase activity-dependent manner; and (ii) indirect regulation of Tbx21 expression through Jmjd3 and T-bet complex formation. Direct regulation of Tbx21 expression by Jmjd3 is consistent with a recent report showing that decreased Tbx21 methylation enhanced Th1 differentiation in Ezh2 -deficient T cells [17] . Further investigation of the mechanistic details by which Jmjd3 binds to the Tbx21 gene promoter to regulate Tbx21 expression is needed. Our study shows that demethylation of H3K27me3 by Jmjd3 is required for optimal T-cell differentiation. Other studies have shown that Jmjd3 functions as a demethylase to control mesodermal and cardiovascular differentiation of mouse embryonic stem cells [50] and M2 macrophage differentiation [37] , [38] . Furthermore, TGF-β-activated Smad2/3 proteins activate target gene expression by recruiting Jmjd3 to counteract Polycomb-mediated repressive H3K27me3 marks [35] . Stat4 recruits Jmjd3 to Th1 genes and affects the production of IFN-γ [51] . In contrast, Jmjd3 regulated T-bet target genes, including Ifng and Cxcr3 , by promoting general chromatin accessibility in a demethylase activity-independent manner [40] . Recently, Jmjd3 was reported to regulate the expression of target genes, including Cxcr3 and Cd44 , through a combination of demethylase-dependent and -independent mechanisms. Some genes, with less H3K27 methylation in the absence of Jmjd3, may have been modulated because of a functional change in UTX ( Kdm6A gene) or Ezh2. Jmjd3 controlled the transcriptional activity of poised RNA polymerase II by demethylating H3K27me3 and interacting with the transcription elongation factors, STP6, IWS1, SETD2 and CHD7 (ref. 52 ). Our findings are in agreement with a previous study demonstrating the requirement for Jmjd3 in RNA polymerase II progression through H3K27me3-enriched gene bodies of TGF-β-responsive genes [53] . Jmjd3 is a H3K27 demethylase without specific DNA-binding properties, and the mechanisms by which it regulates specific gene expression remain unknown. We found that Jmjd3 selectively regulates target gene expression through interactions with transcription factors and epigenetic proteins. Our study provides compelling evidence that in T cells, Jmjd3 specifically interacts with the key transcription factor, T-bet and Ash2L, a core protein of the H3K4 methyltransferase complex. Consistent with our findings, previous studies have shown that Jmjd3 interacts with T-bet and another key component of the H3K4 methyltransferase complex, RbBP5, to regulate the expression of T-bet-dependent target genes, including Ifng and Cxcr3 (refs 39 , 40 ). Although we found that Jmjd3 does not directly interact with RbBP5, it may be required for the T-bet–RbBP5 interaction, because Jmjd3 deficiency disrupted the endogenous T-bet–RbBP5 interaction in T cells and diminished the ability of T-bet to bind to the promoter and gene body regions of Ifng and Cxcr3 . Therefore, our results suggest that Jmjd3 binds to T-bet/RbBP5 and Ash2L to form a stable complex capable of binding to specific gene promoters. Consistent with these findings, Jmjd3 deficiency resulted in a downregulation of CXCR3 expression in T cells. In addition to T-bet and Ash2L, Jmjd3 may interact with other factors, ensuring target gene specificity. Optimal T-bet-dependent gene expression required the Jmjd3-mediated interaction between T-bet and the chromatin remodelling factor, Brg1 (ref. 40 ). Further studies are needed to identify other key transcription factors that interact and act in concert with Jmjd3 to regulate target gene expression. This study is the first, to the best of our knowledge, to provide genetic evidence that Jmjd3 is required for CD4 + T-cell differentiation in vitro and in vivo . These effects of Jmjd3 are mediated through the epigenetic regulation of T cell-related differentiation and transcription factors. Thus, our findings provide new insights into the role and molecular mechanism of action of Jmjd3 in CD4 + T-cell differentiation. Based on our data, we propose a working model by which Jmjd3 regulates CD4 + T-cell differentiation ( Fig. 8d ). In this model, transcription factors, via Ash2L, recruit Jmjd3 interacting with a H3K4 methyltransferase complex, and then the transcription factor physically interacts with a protein within the H3K4 methyltransferase complex, such as RbBP5 or Ash2L. This forms a stable complex capable of binding to target gene promoters, allowing Jmjd3 to alter H3K27 methylation level and RbBP5 and Ash2L to alter H3K4 methylation level to control target gene expression. Jmjd3 upregulates Th1 and Treg cell differentiation factor expression, including Foxp3 , Ifng , Cd44 and Cxcr3 , and downregulates the expression of Th2 and Th17 differentiation factors, including Gata3 and Rorc . These Jmjd3-mediated gene expression changes lead to the promotion of Th1 and Treg cell differentiation and the inhibition of Th2 and Th17 cell differentiation. Mice Jmjd3 flox/flox ( Jmjd3 f/f ) mice were generated by targeting exons 15–21 (encoding the JmjC-catalytic domain) using a Cre-LoxP system. Eight-week-old Jmjd3 f/f male mice were crossed with eight-week-old CD4-Cre female mice (Taconic) to generate Jmjd3 cKO mice. C57BL/6 and 2D2 mice were obtained from the Jackson Laboratory. Rag2 −/− γc −/− mice were purchased from Taconic. Foxp3-GFP reporter mice were kindly provided by Dr Alexander Rudensky (Memorial Sloan-Kettering Cancer Center). All mice were rederived by standard embryo transfer and maintained in pathogen-free animal facilities at Baylor College of Medicine and the Houston Methodist Research Institute. This study was reviewed and approved by Institutional Animal Care and Use Committee at Baylor College of Medicine and the Houston Methodist Research Institute. Splenocyte purification and CD4 + T-cell differentiation Mouse splenocytes were isolated using a negative selection kit (StemCell) and stained for CD4 (anti-CD4-PE, GK1.5, BioLegend; 1:100 dilution), CD25 (anti-CD25-eFluo450, eBioscience, 48-0251-82, 1:100 dilution), CD44 (anti-CD44-APC-eFluo780, clone IM7, eBioscience, 1:100 dilution) and CD62L (anti-CD62L-FITC, eBioscience, 11-0621-85, 1:100 dilution). Naïve CD4 + (CD4 + CD25 - CD44 low CD62L + ) cells were sorted by BD FACSAria II to >95% purity. For in vitro activation, CD4 + T cells were stimulated with 0.5 μg ml −1 soluble anti-CD3 and 1 μg ml −1 anti-CD28 in the presence of 3,000 rads-irradiated T cell-depleted splenocytes as antigen-presenting cells. RPMI medium was supplemented with 10% fetal calf serum, L -glutamine (2 mM), 2-mercaptoethanol (55 μM), penicillin (50 U ml −1 ), streptomycin (50 mg ml −1 ), sodium pyruvate (1 mM) and HEPES (25 mM). Conditions for CD4 + T-cell differentiation were as follows: Th1 cells, IL-12 (10 ng ml −1 )+IL-2 (60 IU ml −1 ); Th2 cells, IL-4 (10 ng ml −1 )+IL-2 (60 IU ml −1 ); Th17 cells, recombinant human (rh)TGFβ1 (5 ng ml −1 )+IL-6 (20 ng ml −1 ); and Treg cells, rhTGFβ1 (5 ng ml −1 )+IL-2 (60 IU ml −1 ). Isolation of intestinal lymphocytes Mice were killed and intestines were removed and placed in ice-cold PBS. After removal of residual mesenteric fat tissue, Peyer’s patches were carefully excised, and the intestine was opened longitudinally. The intestine was thoroughly washed in ice-cold PBS and cut into 0.3–0.5 cm pieces. The pieces were incubated in 20 ml of 2 mM EDTA in 10% fetal bovine serum/PBS for 20 min at 37 °C with slow rotation. After incubation, the epithelial cell layer was removed by intensive vortexing and was passed through a 70-μm cell strainer. The pieces were washed once with PBS, and placed in 20 ml of digestion solution containing 10% fetal bovine serum and 0.5 mg ml −1 of Collagenase IV (Sigma). Digestion was performed by incubating the pieces at 37 °C for 60 min with slow rotation. After the initial 60 min, the solution was vigorously vortexed and passed through a 40-μm cell strainer. The pieces were collected and placed into fresh digestion solution, and the procedure was repeated a total of two times. Supernatants from both digestions were combined, centrifuged and washed once in PBS. The cells were resuspended in 44% (vol/vol) Percoll (GE Healthcare Bio-Sciences), overlaid on 5 ml of 67% Percoll in a 15-ml Falcon tube and centrifuged for 20 min at 625 g at room temperature. Lamina propria lymphocytes were collected at the interphase of the Percoll gradient, washed twice and used immediately for experiments [54] . Flow cytometry and ELISA For detection of surface molecules, T cells were first incubated with an anti-Fc receptor Ab (24G2) to reduce the nonspecific binding of the monoclonal antibodies (mAbs), and then labelled with the appropriate fluorescent mAbs. For the analysis of intracellular cytokine production, T cells were stimulated with phorbol 12-myristate 13-acetate (50 ng ml −1 ) and ionomycin (1 μg ml −1 ) for 4 h in the presence of Golgi Stop solution (BD Biosciences). Cells were collected, washed, fixed, permeabilized (FIX AND PERM, Invitrogen), and stained with fluorescein-labelled cytokine-specific mAbs according to the manufacturer’s instructions. Appropriate fluorescein-conjugated, isotype-matched mAbs were used as negative controls. Cells were analysed using the BD FACS Aria II. IFN-γ and IL-4 production were determined using ELISA kits (R&D Systems) according to the manufacturer’s protocols. In vivo differentiation of naïve CD4 + T cells For long-term T-cell differentiation, a CD4 + T cell-dependent colitis model was used. Naïve CD4 + T cells (CD4 + CD25 - CD62L + CD44 low ) and Treg cells (CD4 + CD25 + ) from eight-week-old WT and Jmjd 3 cKO female mice were purified by FACS, resuspended by gently mixing, and i.p. injected into sublethally irradiated eight-week-old Rag2 −/− γc −/− female mice (1 × 10 6 T cells, or 1 × 10 6 T cells+0.2 × 10 6 Treg cells per mouse). Two weeks later, treated mice were monitored daily for disease progression based on body weight loss, and T-cell subsets in the spleen and intestines were determined at day 29 and day 40 after T-cell transfer. The intestinal inflammation was scored based on: the affected tissue area; the epithelial hyperplasia and goblet cell deficiency; leukocyte infiltration in the lamina propria and the appearance of inflammation markers, including submucosal inflammation and crypt abscesses. For short-term in vivo differentiation, naïve CD4 + T cells (CD4 + CD25 − CD62L + CD44 low ) from eight-week-old WT and Jmjd 3 cKO female mice were intravenously injected into sublethally irradiated eight-week-old Rag2 −/− γc −/− female mice (250 rads). On day 10 after adoptive transfer of naïve CD4 + T cells, spleens were removed and splenocytes were prepared for determination of various CD4 + T-cell subsets by FACS analysis. RNA preparation, RT–PCR and qPCR Total RNAs were isolated from T cells with Trizol reagent (Invitrogen). A total of 0.5 μg of RNA was converted to cDNA using SuperScript III Reverse Transcriptase (Qiagen) with random hexamer primers. qPCR was performed using the ABI Prism 7000 Analyzer (Applied Biosystems) with SYBR Green mix (Applied Biosystems). All primers are listed in Supplementary Table 2 . Immunoblotting analysis Cells were collected and lysed in RIPA buffer with protease inhibitors and 2 μM phenylmethylsulphonyl fluoride. Protein extracts were boiled in SDS sample buffer for 5 min, loaded directly onto a 4–12% SDS gel, transferred onto nitrocellulose membranes (Bio-Rad), blocked with 5% milk and incubated with corresponding primary and secondary antibodies using standard protocols. The following antibodies were used: anti-H3K4me1 (Cat # 07-436, 1:2,000 dilution), anti-H3K4me2 (Cat # 07-030, 1:4,000 dilution), anti-H3K4me3 (Cat # 07-473, 1:4,000 dilution), anti-H3K9me1 (Cat # 07-450, 1:2,000 dilution), anti-H3K9me2 (Cat # 07-441, 1:3,000 dilution), anti-H3K9me3 (Cat # 07-442, 1:3,000 dilution), anti-H3K27me1 (Cat # 07-448, 1:2,000 dilution), anti-H3K27me2 (Cat # 07-452, 1:4,000 dilution) and anti-H3K27me3 (Cat # 07-449, 1:4,000 dilution) from Millipore; rabbit anti-Jmjd3 (Cat # ab1022a, 1:500 dilution) from Abgent; and mouse anti-FLAG (1:5,000 dilution), anti-HRP-FLAG (1:5,000 dilution) and anti-β-actin (1:5,000 dilution) from Sigma; anti-Smad1 (Cat # 6944, 1:500 dilution), anti-Smad2 (Cat # 5339, 1:500 dilution) and anti-Smad3 (Cat # 9523, 1:500 dilution) from Cell Signaling; and anti-Ash2L (Cat # ab50699, 1:500 dilution) from Abcam. ChIP-Seq and ChIP-PCR analyses A total of 200 ng of DNA from WT and Jmjd3 cKO CD4 + T cells was used for the ChIP-Seq library construction. Illumina sequencing was performed according to previously described protocols [44] , [55] , [56] . Sequencing reads from H3K4me3 and H3K27me3 ChIP-Seq libraries were aligned to the mouse mm8 genome using ELAND software. To reduce PCR amplification bias, only one uniquely mapped read per genomic position was retained. The histone modification changes upon Jmjd3 knockout were assessed as follows. The H3K27me3 sequencing reads in WT and cKO samples were counted in 4 kb windows centred at TSS or p300 ChIP-Seq peaks. The resulting read counts were used as input to the DEGseq algorithm [56] to identify differentially methylated genes and enhancers. The DEGseq q -value cutoff of 0.05 and the fold-change cutoff of 2 were used to identify statistically significant methylation changes. The GEO (Gene Expression Omnibus) accession number for the raw and analysed ChIP-seq data is GSE58775. ChIP-PCR experiments were performed using the Imprint Chromatin Immunoprecipitation Kit (Sigma) according to the manufacturer’s instructions. All primers are listed in Supplementary Table 2 . Statistical analysis Data are reported as the mean±standard deviation (s.d.) where indicated. Differences between groups were analysed using the Student’s t -test with GraphPad Prism 4.0 software. A P value <0.05 was considered statistically significant. How to cite this article: Li, Q. et al . Critical role of histone demethylase Jmjd3 in the regulation of CD4 + T-cell differentiation. Nat. Commun. 5:5780 doi: 10.1038/ncomms6780 (2014).